Protein-pyridinol thioester precursor for biosynthesis of the organometallic acyl-iron ligand in [Fe]-hydrogenase cofactor The iron-guanylylpyridinol (FeGP) cofactor of [Fe]-hydrogenase contains a prominent iron centre with an acyl-Fe bond and is the only acyl-organometallic iron compound found in nature. Here, we identify the functions of HcgE and HcgF, involved in the biosynthesis of the FeGP cofactor using structure-to-function strategy. Analysis of the HcgE and HcgF crystal structures with and without bound substrates suggest that HcgE catalyses the adenylylation of the carboxy group of guanylylpyridinol (GP) to afford AMP-GP, and subsequently HcgF catalyses the transesterification of AMP-GP to afford a Cys (HcgF)-S-GP thioester. Both enzymatic reactions are confirmed by in vitro assays. The structural data also offer plausible catalytic mechanisms. This strategy of thioester activation corresponds to that used for ubiquitin activation, a key event in the regulation of multiple cellular processes. It further implicates a nucleophilic attack onto the acyl carbon presumably via an electron-rich Fe(0)– or Fe(I)–carbonyl complex in the Fe-acyl formation. Nature expands the catalytic capability of proteins by developing metal cofactors [1] . Some of the most attractive representatives are those of [NiFe]-, [FeFe]- and [Fe]-hydrogenases, which catalyse the production and consumption of H 2 in microorganisms [2] , [3] , [4] , [5] . The unusual Fe centres of [NiFe]- and [FeFe]-hydrogenases contain thiolate, CO and CN − ligands. Instead of CN − ligands, the Fe centre of the iron-guanylylpyridinol (FeGP) cofactor of [Fe]-hydrogenase has a guanylylpyridinol (GP), which is bidentately chelated to Fe by its nitrogen and acyl-carbon [6] , [7] . The Fe-acyl bond constitutes the only stable acyl-organometallic compound found in nature, although an acyl-Ni species has been reported to be an intermediate in the acetyl-CoA formation reaction catalysed by acetyl-CoA synthase [8] , [9] . The metal cofactors of hydrogenases and their biosynthesis have been extensively explored to unravel their fascinating chemistry [10] , [11] , [12] and to use their H 2 activation capabilities for biotechnological applications [13] , [14] . In contrast to studies of [NiFe]- and [FeFe]-hydrogenases, convincing hypotheses and experimental data have not been reported for the biosynthesis of the Fe centre of [Fe]-hydrogenase, including the formation of the unique acyl-group, the greatest challenge in FeGP cofactor biosynthesis. The seven conserved hmd co-occurring ( hcgA - G ) genes in the genomes of hydrogenotrophic methanogens are involved in the biosynthesis of the FeGP cofactor [15] , [16] . Recent findings using structure-to-function strategy [17] , [18] indicated that the formation of 6-carboxymethyl-guanylylpyridinol from GTP and a pyridinol compound are catalysed by HcgB, which strongly suggested that GP is an intermediate in the FeGP biosynthetic pathway and, consequently, that its carboxy group is converted to the acyl-iron ligand in subsequent enzymatic reactions [19] . In the current study, we find that HcgE and HcgF catalyse the formation of a thioester-activated acyl-group using a two-state mechanism reminiscent of that of ubiquitin activation [20] . HcgE catalyses the adenylylation of the carboxy group of GP to afford adenosine 5′-monophosphate (AMP)-GP. HcgF catalyses the transesterification of AMP-GP to afford a Cys-S-GP thioester. On the basis of the findings, possible Fe-acyl formation mechanisms are proposed. Structural identification of substrates of HcgE The functional characterization of HcgE was inspired by the relationship between the primary structures of HcgE and E1-like ubiquitin-activating enzymes (E1 enzymes) ( Supplementary Figs 1 and 2 ) [20] . E1 enzymes activate the C-terminal carboxy group of ubiquitin or ubiquitin-like proteins and of a precursor heptapeptide of an antibiotic by adenylylation with adenosine 5′-triphosphate (ATP). This essential activation reaction is performed by various eukaryotic E1 enzymes/ubiquitin-like proteins [20] , [21] , and by the prokaryotic protein pairs MoeB/MoaD [22] , ThiF/ThiS [23] and MccB/MccA [24] , which are involved in the modulation of protein function in the regulation of multiple cellular processes and in the biosynthesis of molybdopterin, thiamine and the antibiotic microcin C7, respectively. Likewise, HcgE might therefore catalyse the adenylylation of a carboxy group of an unknown compound, that is, GP, in FeGP cofactor biosynthesis. Structures of [Fe]-hydrogenase, the FeGP cofactor and GP are shown in Fig. 1 . 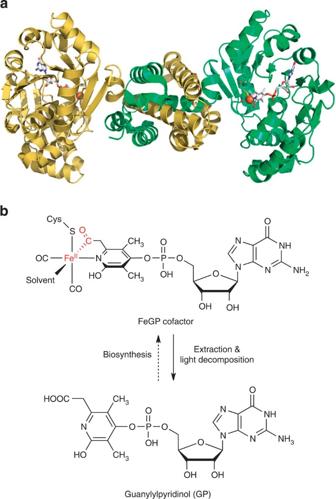Figure 1: [Fe]-hydrogenase and FeGP cofactor. (a) Crystal structure of dimeric [Fe]-hydrogenase with bound FeGP cofactor shown as a ball-and-stick model. This enzyme is involved in the methanogenic energy metabolism of many hydrogenotrophic methanogens. (b) Biosynthesis and light decomposition of the FeGP cofactor. The FeGP cofactor can be extracted with methanol in the presence of 2-mercaptoethanol and decomposed by light exposure to Fe2+, CO and GP, in which the acyl-group is hydrolysed to a carboxy group34. GP appears to be a natural intermediate in the FeGP cofactor biosynthesis pathway of the cells19. An acyl-iron bond (red) is only found in the FeGP cofactor. Figure 1: [Fe]-hydrogenase and FeGP cofactor. ( a ) Crystal structure of dimeric [Fe]-hydrogenase with bound FeGP cofactor shown as a ball-and-stick model. This enzyme is involved in the methanogenic energy metabolism of many hydrogenotrophic methanogens. ( b ) Biosynthesis and light decomposition of the FeGP cofactor. The FeGP cofactor can be extracted with methanol in the presence of 2-mercaptoethanol and decomposed by light exposure to Fe 2+ , CO and GP, in which the acyl-group is hydrolysed to a carboxy group [34] . GP appears to be a natural intermediate in the FeGP cofactor biosynthesis pathway of the cells [19] . An acyl-iron bond (red) is only found in the FeGP cofactor. Full size image To experimentally explore this hypothesis, we determined the crystal structure of homotrimeric HcgE and of the HcgE–ATP complexes from Methanothermobacter marburgensis ( Fig. 2a ; Supplementary Figs 3 and 4 ) at 1.6 and 1.8 Å resolution, respectively. ATP binds to the canonical ATP-binding site of E1 enzymes located in the conserved N-terminal half. In contrast, the fold of the C-terminal half substantially differs between HcgE and the structurally known E1 enzymes, resulting in a completely altered substrate-binding site ( Fig. 2b ; Supplementary Fig. 3 ). We identified GP as a possible substrate of HcgE on the basis of the ternary HcgE–ATP–GP complex structure determined at 2.8 Å resolution ( Fig. 2c,d ). Notably, GP binding was only achievable when HcgE and GP were crystallized in the presence of ATP. Despite different substrate-binding sites, the carboxy group of GP in HcgE and the carboxy group of the C-terminal glycine of MoaD are in equivalent position. 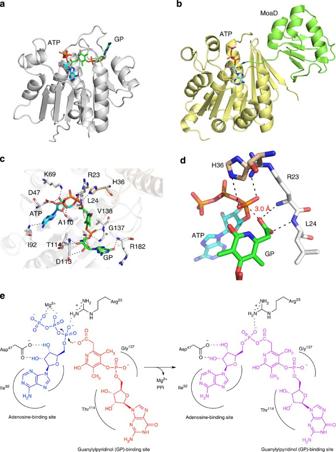Figure 2: Crystal structure and mechanism of HcgE. (a) Structure of HcgE (grey) in complex with ATP (carbon in cyan) and GP (carbon in green). (b) Structure of MoeB (yellow) with ATP (carbon in cyan) and MoaD (green)22. The ATP-binding site of HcgE and MoeB are conserved, whereas their GP- and MoaD-binding sites but not the position of their corresponding carboxy group markedly vary. (c) The ATP- and GP-binding sites. ATP is present in a hairpin-like and GP in a slightly bent conformation. Polar interactions are indicated as black dashed lines. (d) Transition state-like arrangement of GP and ATP. The carboxy group of GP points to the α-phosphate of ATP. The distance between the oxygen atom of the carboxy group of GP and the phosphorus atom of the α-phosphate group of ATP is shown as a red dashed line. (e) Mechanism proposed for the HcgE-catalysed adenylylation of GP with ATP. Figure 2: Crystal structure and mechanism of HcgE. ( a ) Structure of HcgE (grey) in complex with ATP (carbon in cyan) and GP (carbon in green). ( b ) Structure of MoeB (yellow) with ATP (carbon in cyan) and MoaD (green) [22] . The ATP-binding site of HcgE and MoeB are conserved, whereas their GP- and MoaD-binding sites but not the position of their corresponding carboxy group markedly vary. ( c ) The ATP- and GP-binding sites. ATP is present in a hairpin-like and GP in a slightly bent conformation. Polar interactions are indicated as black dashed lines. ( d ) Transition state-like arrangement of GP and ATP. The carboxy group of GP points to the α-phosphate of ATP. The distance between the oxygen atom of the carboxy group of GP and the phosphorus atom of the α-phosphate group of ATP is shown as a red dashed line. ( e ) Mechanism proposed for the HcgE-catalysed adenylylation of GP with ATP. Full size image In vitro activity assay of HcgE To complement the structure-guided functional prediction, we analysed a reaction mixture containing HcgE, ATP, GP and Mg 2+ by matrix-assisted laser desorption/ionization time-of-flight mass spectrometry (MS) ( Supplementary Fig. 5 ). The obtained peak at m/z 872.2 corresponded to the expected product AMP-GP (calculated mass=871.2) and its fragmentation peaks at m/z 348.1 and 525.1 corresponded to AMP and GP, respectively. HcgE activity followed Michaelis–Menten kinetics with an apparent K m for ATP of 27.0±3.5 μM and a k cat of 7.2±0.2 min −1 based on determination of the pyrophosphate concentration ( Supplementary Fig. 6 ). Thus, structural, mass spectrometry and kinetic data identified HcgE as an adenylyltransferase that forms AMP-GP from ATP and GP. Catalytic mechanism of HcgE The ternary structure of the HcgE–ATP–GP complex revealed that the carboxy group of GP points towards the α-phosphate group of ATP ( Fig. 2c,d ). This transition state-like arrangement not only strongly argues for an adenylylation reaction catalysed by HcgE but also provides clues to its catalytic mechanism ( Fig. 2e ). In this proposed mechanism, the carboxy group of GP attacks the α-phosphate of ATP via an S N 2 reaction thereby adenylylating GP via a pentavalent intermediate. The negative charge of the carboxy oxygen of GP is compensated by a hydrogen bond to Leu24-NH located at the N-terminal side of helix 24:34. The guanidinium group of Arg23 and the imidazole group of His36 of the partner subunit of the trimer compensate the negative charge of the α-phosphate oxygen of ATP ( Fig. 2c,d ). The negative charge of the released pyrophosphate is delocalized by interactions with Mg 2+ (not visible in the electron density map), which probably interacts with its β- and γ-phosphates and with several polypeptide side chains ( Fig. 2e ). Possible function of HcgF provided by protein structure We determined the function of HcgF using the structure-to-function strategy used for HcgE. HcgF does not show sequence similarities to any enzyme of known function ( Supplementary Figs 7 and 8 ), but the crystal structure determined for homodimeric HcgF from Methanocaldococcus jannaschii is strongly related to that of the nicotinamide mononucleotide (NMN) deaminase PncC [25] ( Supplementary Fig. 9 ). HcgF does not exhibit NMN hydrolase activity, but the profiles of the proposed NMN-binding cavity of PncC and the equivalent site of HcgF are compatible with the demands for accommodating an NMN-like compound, that is, GP ( Supplementary Fig. 9 ). Indeed, the X-ray crystal structure of HcgF at 2.0 Å resolution co-crystallized with GP revealed bound GP ( Fig. 3a–d ). Interestingly, GP in one HcgF monomer of the asymmetric unit partially forms a covalent thioester bond between its carboxy carbon and the thiolate of Cys9 ( Fig. 3c,d ), while in the other monomer, Cys9 and GP are in van der Waals contact ( Fig. 3b ; Supplementary Fig. 10 ). In the substrate-free HcgF, the strictly conserved Cys9 is activated by the neighbouring Lys79-N. Upon binding of GP, conformational changes of the segments after strands 46:53 and 125:131 up to 6 Å enlarge the substrate-binding site and, concomitantly, induce a movement of the side chain of Lys79 by more than 10 Å from the largely buried Cys9 towards the protein surface ( Fig. 3b,c ). The key residue Cys9 positioned at the C-terminal end of the shortened strand 4:9 is strictly conserved in HcgF. 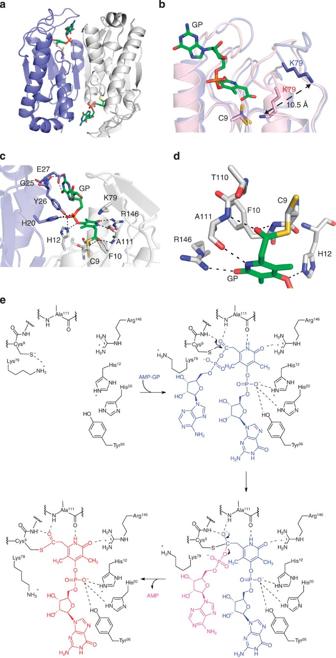Figure 3: Crystal structure and catalytic mechanism of HcgF. (a) Structure of HcgF in complex with GP (green). In the two active sites of the homodimer, the Cys9 sulfur and the GP acyl carbon either contact each other or partially form a covalent bond. (b) Superimposed structures of GP-free (light magenta) and non-covalently GP-bound HcgF (blue). Cys9 is presumably kept in the more reactive thiolate form by Lys79 in the resting state and attacks activated GP (green) after its binding. (c) The GP-binding site with GP covalently bound to Cys9. (d) The thioester bond between GP and Cys9. The extra S (yellow) indicates the second conformation of the Cys9 side chain. (e) Proposed catalytic mechanism of the thioester formation of AMP-GP with Cys9 of HcgF. Figure 3: Crystal structure and catalytic mechanism of HcgF. ( a ) Structure of HcgF in complex with GP (green). In the two active sites of the homodimer, the Cys9 sulfur and the GP acyl carbon either contact each other or partially form a covalent bond. ( b ) Superimposed structures of GP-free (light magenta) and non-covalently GP-bound HcgF (blue). Cys9 is presumably kept in the more reactive thiolate form by Lys79 in the resting state and attacks activated GP (green) after its binding. ( c ) The GP-binding site with GP covalently bound to Cys9. ( d ) The thioester bond between GP and Cys9. The extra S (yellow) indicates the second conformation of the Cys9 side chain. ( e ) Proposed catalytic mechanism of the thioester formation of AMP-GP with Cys9 of HcgF. Full size image AMP-GP is the substrate of HcgF Consideration of the obtained structural data and the established reaction of HcgE led to the proposal that the same two-step carboxylate activation strategy reported for ubiquitin activation is used in the biosynthesis of the FeGP cofactor, namely adenylylation of the carboxy group of GP by HcgE, followed by thioester formation by HcgF ( Fig. 4 ). This hypothesis implies that not GP but rather AMP-GP formed by the HcgE reaction is the natural substrate of HcgF. Unfortunately, the instability of AMP-GP, precludes its use in crystallographic studies. Docking simulation of AMP on GP covalently bound to HcgF, however, indicated that it is spatially possible for AMP-GP to be accommodated in the binding site adjacent to Cys9 ( Supplementary Fig. 9c ). To demonstrate the transesterification reaction from AMP-GP to Cys9 (HcgF)-GP in solution, we added HcgF to the HcgE reaction assay described above. The production of AMP confirmed the proposed function of HcgF ( Supplementary Fig. 11 ). 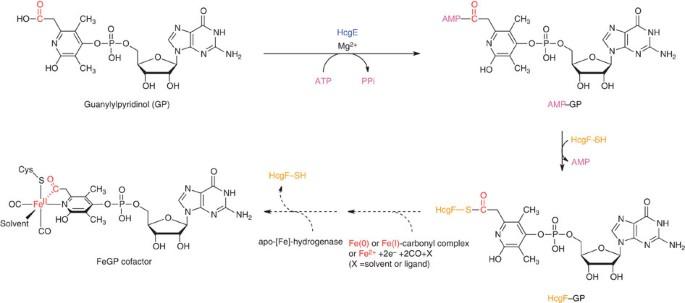Figure 4: A proposed biosynthetic pathway to the FeGP cofactor. The carboxy group of GP is adenylated by HcgE using ATP and Mg2+to form AMP-GP; released AMP-GP is bound by HcgF and forms a covalent HcgF-GP thioester adduct with the Cys9 thiolate; and the reactive thioester between GP and HcgF is converted to an acyl-Fe bond perhaps by a nucleophilic substitution of an electron-rich Fe from an unknown iron–carbonyl precursor. The thiolate of Cys9 of HcgF is an excellent leaving group, especially when its negative charge is compensated by protonation or hydrogen-bond interactions. Figure 4: A proposed biosynthetic pathway to the FeGP cofactor. The carboxy group of GP is adenylated by HcgE using ATP and Mg 2+ to form AMP-GP; released AMP-GP is bound by HcgF and forms a covalent HcgF-GP thioester adduct with the Cys9 thiolate; and the reactive thioester between GP and HcgF is converted to an acyl-Fe bond perhaps by a nucleophilic substitution of an electron-rich Fe from an unknown iron–carbonyl precursor. The thiolate of Cys9 of HcgF is an excellent leaving group, especially when its negative charge is compensated by protonation or hydrogen-bond interactions. Full size image Catalytic mechanism of HcgF A proposed reaction mechanism for the thioester bond formation between Cys9 of HcgF using AMP-GP as a substrate is shown in Fig. 3e . In this mechanism, the thiolate of Cys9 attacks the adenylated carboxy group of AMP-GP in a S N 2 reaction, resulting in the formation of a thioester bond and the release of AMP. The oxygen of the thioester group interacts with Phe10-NH and Ala111-NH (see also Fig. 3d ), which most likely also stabilizes the anionic tetrahedral transition state. Notably, the GP-HcgF adduct is the first example of a ubiquitin activation system for which the thioester product has been structurally characterized. The identified GP carboxylate activation involved in Fe-acyl formation corresponds to the mechanism established for ubiquitin activation and thereby expands this versatile strategy from (poly)peptides to other carboxylated substrates. Activation via a thioester bond suggests a nucleophilic substitution reaction for Fe-acyl formation to allow the release of Cys9 (HcgF) as thiolate, which is a favourable leaving group ( Fig. 4 ). An iron–carbonyl precursor, so far uncharacterized in the biosynthesis of the [Fe]-hydrogenase cofactor but experimentally identified in that of [NiFe]- and [FeFe]-hydrogenase [11] , [26] , [27] , can in principle, provide a nucleophilic iron as central atom. An Fe(0)–carbonyl complex as the precursor of acyl-iron ligand biosynthesis appears to be suitable and has been used for chemical synthesis of the Fe-acyl bond of FeGP cofactor model compounds [28] . However, the formation of an Fe(0)–carbonyl complex precursor requires a chemistry challenging in a water-rich biological environment, such as that of the novel iron(II)-complex reduction system in methanogenic archaea ( Fig. 4 ). Alternatively, a one-electron reduction system might formally generate a Fe(I)–carbonyl complex for nucleophilic attack, followed by a second one-electron reduction step such as proposed for the catalytic mechanism of acetyl-coenzyme A synthase [8] . The enzymatic system involved in the Fe-acyl formation is unknown. HcgF could also function as a scaffold protein on which biosynthesis of the FeGP cofactor is completed after an electron-rich Fe–carbonyl complex is accepted. The intact cofactor biosynthesized on HcgF could be transferred to the [Fe]-hydrogenase apoenzyme to form its holoenzyme. However, a scaffold function of the other enzymes cannot be excluded [17] , [29] . Nevertheless, the established thioester activation offers first insights into the chemistry of the subsequent Fe-acyl bond formation and places this reaction in the pathway of Fe centre biosynthesis after iron–carbonyl formation. Chemicals All chemicals were used without further purification. ATP, AMP, ammonium acetate, pentaerythritol ethoxylate 270 (3/4 EO/OH), (±)-2-methyl-2,4-pentanediol, nickel sulphate, potassium hydroxide, lithium sulphate, thrombin from bovine plasma and inorganic pyrophosphatase from Saccharomyces cerevisiae were purchased from Sigma-Aldrich. L -(+)-Selenomethionine (SeMet) was purchased from Acros Organics. Magnesium chloride, PEG6000, PEG3000 and thiamine were purchased from Merck. The following reagents were obtained from Roth: acetonitrile, kanamycin sulphate, 3-( N -morpholino)propanesulfonic acid (MOPS), 4-(2-hydroxyethyl)piperazine-1-ethanesulfonic acid (HEPES), 2-( N -morpholino)ethanesulfonic acid (MES), imidazole, ammonium sulphate, ammonium chloride, sodium acetate, sodium chloride, sodium citrate, hydrochloric acid, potassium chloride, potassium dihydrogen phosphate, dipotassium hydrogen phosphate, dithiothreitol (DTT), D-(+)-glucose, FeCl 3 ·6H 2 O. Isopropyl β- D -thiogalactopyranoside (IPTG) was purchased from Fermentas and Pi ColorLock Gold for quantification of inorganic monophosphate from Innova Biosciences. The FeGP cofactor was extracted from [Fe]-hydrogenase from M. marburgensis in a solution containing 60% methanol, 1 mM 2-mercaptoethanol and 1% ammonia and then purified with Q-Sepharose and G25 columns [29] , [30] . GP was generated by irradiation of the extracted FeGP cofactor with room light under N 2 and then purified using HPLC with 6 ml Resource Q column (GE Healthcare) and further purified with Synergi 4 μ Polar RP 80 A column (250 × 4.6 mm, Phenomenex) [30] . The M. marburgensis hcgE gene and the M. jannaschii hcgF gene with codon optimization for Escherichia coli host cells were purchased from GenScript USA Inc as hcgE -pET24b (Novagen) and hcgF -pET28b (Novagen) plasmids, respectively. The synthesized M. marburgensis hcgE gene encoded a thrombin cleavage site and a His 6 -tag at its 3′ end. Heterologous production and purification of HcgE The synthesized M. marburgensis hcgE gene ( Supplementary Fig. 12 ) inserted into the Nde I and Sal I sites of pET24b plasmid was introduced into E. coli BL21 (DE3) (Agilent Technologies) by transformation. The transformed cells were incubated in LB medium containing 50 μg ml −1 kanamycin at 37 °C to an optical density (OD) 600 of 1.0. Gene expression was induced by addition of 0.5 mM IPTG. After further incubation for 4–6 h, the cells were harvested by centrifugation and stored at −80 °C until use. The frozen cells were resuspended in a solution of 50 mM potassium phosphate, pH 7.0, 0.5 M KCl and 20 mM imidazole (buffer A) and were disrupted by sonication. The supernatant was collected after centrifugation and loaded onto a Ni 2+ -charged HiTrap chelating column (GE Healthcare) equilibrated with buffer A. The column was washed with 15 column volumes of buffer A and eluted with a linear gradient of imidazole from 20 to 500 mM in 50 mM potassium phosphate, pH 7.0, with 0.5 M KCl. After the fractions containing C-terminal His 6 -tagged HcgE protein were pooled and concentrated, the protein solution was loaded onto a HiPrep 26/10-desalting column (GE Healthcare) equilibrated with 50 mM potassium phosphate, pH 7.0, containing 0.3 M KCl. After desalting, the protein fraction was incubated with thrombin (10 units per mg HcgE) at 4 °C overnight to cleave the His 6 -tag. The His 6 -tag and thrombin were then removed on a Ni 2+ -charged HiTrap chelating column and a HiTrap Benzamidine FF column (GE Healthcare) equilibrated with buffer A, and eluted with a linear gradient of KCl from 0.5 to 2.0 M in 50 mM KPi buffer (pH 7.0) containing 20 mM imidazole. After fractions containing the HcgE protein were pooled and concentrated, the protein solution was loaded onto a Sephacryl S-200 column (GE Healthcare) equilibrated with 50 mM potassium phosphate, pH 7.0, with 0.3 M KCl and eluted with the same buffer as used for the equilibration. Heterologous production and purification of HcgF The synthesized M. jannaschii hcgF gene ( Supplementary Fig. 13 ) inserted into the Nde I and Hin dIII sites of pET28b was introduced into E. coli BL21 (DE3) Star (Invitrogen) by transformation. The transformed cells were grown in LB medium containing 50 μg ml −1 kanamycin at 37 °C to an OD 600 of 1.0. Protein expression was induced by addition of 1.0 mM IPTG and further incubation for 4–6 h. The N-terminal His 6 -tagged HcgF protein was purified, and the His 6 -tag was cleaved as described for the His 6 -tagged HcgE protein. To remove the His 6 -tag and thrombin, the reaction mixture of HcgF and thrombin was loaded onto a Ni 2+ -charged HiTrap chelating column and a HiTrap Benzamidine FF column (GE Healthcare) equilibrated with buffer A. After the fractions containing the HcgF protein were isocratically eluted and concentrated, the protein solution was loaded onto a Sephacryl S-200 column (GE Healthcare) equilibrated with 50 mM potassium phosphate buffer (pH 7.0) containing 0.3 M KCl and eluted with the same buffer as used for the equilibration. For the SeMet-labelled HcgF preparation, E. coli B834 (DE3) (Novagen) cells transformed with pET28b carrying the synthesized M. jannaschii hcgF gene inserted into its Nde I and Hin dIII sites were incubated in M9 medium supplemented with 2.5 mM MgSO 4 , 2% (w/v) D -(+)-glucose, 0.01% (w/v) thiamine, 0.025 mM FeCl 3 , 50 μg ml −1 L-selenomethionine and 50 μg ml −1 kanamycin at 37 °C to an OD 600 of 0.5. SeMet-HcgF was purified as described for HcgF, except that all buffers contained 1 mM DTT. Crystallization of HcgE A 1-μl aliquot of HcgE (12 mg ml −1 ) in 10 mM MOPS/KOH, pH 7.0, was mixed with 1 μl of a reservoir solution composed of 15% (w/v) PEG6000 and 100 mM sodium citrate (pH 5.0). Crystals of HcgE were obtained by sitting-drop vapour diffusion at room temperature within 2 weeks. For co-crystallization of HcgE with ATP, an aliquot of 1 μl of HcgE (19 mg ml −1 ) in 10 mM MOPS/KOH, pH 7.0, was mixed with 0.2 μl of 20 mM ATP and 1.2 μl of a reservoir solution composed of 35% (w/v) pentaerythritol ethoxylate 270 (3/4 EO/OH), 200 mM ammonium sulphate and 100 mM sodium acetate, pH 4.6. Co-crystals of HcgE wtih ATP were obtained by sitting-drop vapour diffusion at room temperature within 1 week. For co-crystallization of HcgE with ATP and GP, a 0.5-μl aliquot of HcgE (30 mg ml −1 ) in 10 mM MOPS/KOH, pH 7.0, was mixed with 0.5 μl of 2.5 mM GP, 0.5 μl of 2.5 mM ATP and 1.5 μl of a reservoir solution composed of 35% (w/v) pentaerythritol ethoxylate 270 (3/4 EO/OH), 200 mM ammonium sulphate and 100 mM sodium acetate, pH 4.6. Crystals of HcgE incubated with ATP and GP were obtained by sitting-drop vapour diffusion at room temperature within 1 week. Crystallization of HcgF A 1-μl aliquot of HcgF (15 mg ml −1 ) in 50 mM MES/KOH, pH 7.0, was mixed with 1 μl of a reservoir solution composed of 20% (w/v) PEG3000, 200 mM NaCl and 100 mM HEPES/KOH, pH 7.5. Crystals of HcgF were obtained by sitting-drop vapour diffusion at room temperature within 2 weeks. For crystallization of SeMet-labelled HcgF, a 1 μl aliquot of SeMet-HcgF (19 mg ml −1 ) in 50 mM MES/KOH, pH 7.0, containing 1 mM DTT was mixed with 1 μl of a reservoir solution composed of 20% (w/v) PEG3000, 200 mM NaCl and 100 mM HEPES-NaOH, pH 7.5. Crystals of SeMet-HcgF were obtained by sitting-drop vapour diffusion at room temperature within 2 weeks. For co-crystallization of HcgF with GP, a 0.5 μl aliquot of HcgF (8.6 mg ml −1 ) in 10 mM MOPS/KOH, pH 7.0, containing 1 mM DTT was mixed with 0.5 μl of 2.5 mM GP and 1 μl of a reservoir solution composed of 40% (v/v) (±)-2-methyl-2,4-pentanediol and 200 mM Li 2 SO 4 . Crystals of HcgF incubated with GP were obtained by sitting-drop vapour diffusion at room temperature within 3 days. X-ray data collection and refinement The crystal of HcgE was immersed into a reservoir solution containing 20% (v/v) ethylene glycol for cryoprotection before freezing the crystal under a cryo-stream of N 2 at 100 K. The crystals of ATP-bound HcgE, ATP-GP-bound HcgE, HcgF, SeMet-labelled HcgF and GP-bound HcgF were frozen under a cryo-stream of N 2 at 100 K without adding a cryoprotectant. Diffraction data were collected on the beamline X10SA equipped with a PILATUS 6 M detector at the Swiss-Light-Source (Villigen, Switzerland) at 100 K. Data were processed using X-ray Detector Software (XDS) [31] . The HcgE structure was solved by molecular replacement with Molrep [32] using a ThiF (PDB code: 1ZUD)-based model created by the Robetta server [33] . Automated model building was then performed by ARP/wARP [34] to model amino-acid fragments and loops of HcgE. ATP-bound and ATP-GP-bound HcgE structures were solved by molecular replacement with Molrep using the solved HcgE structure. The HcgE models after molecular replacement and automated model building were completed and refined using COOT [35] , REFMAC5 (ref. 36 ) and PHENIX [37] . For the HcgE structure, one out of three monomers in the asymmetric unit showed electron density at the equivalent position of ATP in ATP-bound HcgE, although no ligands were added during the crystallization. On the basis of the shape of the density, ADP and not ATP could be fitted. An explanation is that ADP or ADP-like compounds may slightly co-purify with HcgE from E. coli cells. Phenix Xtriage [37] indicated that the data of HcgE co-crystallized with ATP or with both ATP and GP were merohedral twinned with twin fractions of 0.43 and 0.44 and with twin operators of k , h , - l and - h , - k , l ; k , h , - l ; - k , - h , - l , respectively. Twin refinement was performed with Refmac5 in the amplitude-based mode. To determine the crystal structure of HcgF, multiple anomalous dispersion data at the selenium edge of the SeMet-HcgF crystal was measured. Selenium atom sites were detected with SHELX C/D [38] . The selenium sites were refined and the phase was determined using the program SHARP and improved by the solvent-flattening procedure of SOLOMON implemented in SHARP [39] . The electron density after phasing and solvent flattering was shown as a blue mesh contoured at 1σ ( Supplementary Fig. 14 ). Automatic model building was performed using ARP/wARP [34] . GP-HcgF was solved by molecular replacement with Molrep using the solved HcgF structure as a search model. Further modelling and refinement of HcgF and GP-HcgF were performed using COOT, REFMAC5 and PHENIX. The thioesterified GP model was generated by the Dundee Prodrg server [40] . TLS refinement was performed in the final stage of refinement [41] . Structures were validated using MolProbity [42] . Simulated annealing refined 2 F o − F c omit maps for ATP-bound HcgE, ATP-GP-bound HcgE and GP-bound HcgF were calculated using PHENIX ( Supplementary Fig. 15 ). The resulting structures were established at 1.6 Å (HcgE, PDB: 3WV7), 1.8 Å (ATP-bound HcgE, PDB: 3WV8), 2.8 Å (ATP-GP-bound HcgE, PDB: 3WV9), 1.7 Å (HcgF, PDB: 3WVB), 1.4 Å (SeMet-labelled HcgF, PDB: 3WVA) and 2.0 Å (GP-bound HcgF, PDB: 3WVC). Data collection and refinement statistics are summarized in Supplementary Table 1 . All the protein figures were generated using PyMOL (version 1.3r1, Schrödinger, LLC). Search for structural homologues of HcgE and HcgF Structural homologues of HcgE and HcgF were identified with the Dali server [43] using the crystal structure of HcgE and HcgF. Crystal structures of HcgE and HcgF were superimposed on their homologues using the SUPERPOSE program [44] in the CCP4 suite [45] . Sequence comparison of HcgE and HcgF The amino-acid sequences of HcgE and HcgF from M. jannaschii , Methanococcus maripaludis , Methanobrevibacter smithii , M. marburgensis and Methanopyrus kandleri were aligned using Clustal W2 (ref. 46 ). The amino-acid sequence alignments of HcgE with its structural homologues, Schizoscaccharomyces pombe E1 ubiquitin-activating enzyme [47] , E. coli MoaB [22] , E. coli ThiF [48] and E. coli MccB [24] were also performed using the same method. HcgF structural homologues of Agrobacterium fabrum CinA (PDB code: 2A9S) and NMN deamidases, that is, E. coli YgaD, Shewanella oneidensis PncC [25] and Oceanobacillus iheyensis PncC [49] , were also aligned with HcgF from M. jannaschii using Clustal W2. The figures of the alignment were generated using ESPript3 (ref. 50 ). Docking simulation Molecular docking of AMP to the GP-thioester-binding site of HcgF was performed with AutoDock Vina [51] . For docking calculations, an AMP molecule was placed in a pocket adjacent to the GP-binding site. The calculation converged in an orientation of AMP in which its phosphate is close to the carboxy group of GP. In the case of NMN docking to CinA, the NMN molecule was placed close to a NMN-binding site proposed previously [25] . The calculation has converged, and the most probable binding mode of NMN to CinA was selected. Assay for adenylylation of GP catalysed by HcgE The HcgE-catalysed adenylylation reaction of GP was carried out in 1 μM HcgE, 1 μM inorganic pyrophosphatase, 0.25 mM GP, 0–0.25 mM ATP, 1 mM MgCl 2 and 10 mM MOPS/KOH, pH 7.0, at 30 °C for 10 min. The activity of HcgE was determined by analysing the amount of inorganic pyrophosphate released from the HcgE-catalysed reaction; the pyrophosphate was converted to monophosphate by inorganic pyrophosphatase from S. cerevisiae (Sigma-Aldrich Co. LCC. ), and the monophosphate was analysed using Pi ColorLock Gold (Innova Biosciences). The AMP-GP product in the HcgE-catalysed reaction was analysed by matrix-assisted laser desorption time-of-flight MS and MS/MS. Assay for GP-HcgF thioester bond formation The GP-HcgF thioester bond formation was assayed by monitoring the amount of AMP resulting from a plausible reaction of HcgF with AMP-GP that was produced by HcgE-catalysed adenylylation of GP with ATP. The reaction conditions were as follows: 5 mM MgCl 2 , 5 mM ATP, 0.25 mM GP, 27 μM HcgE and 0–49 μM HcgF in 11 mM potassium phosphate, pH 7.0, containing 63 mM KCl and 0.05 mM DTT at 65 °C for 10 min. The AMP amount was analysed with a HPLC system (JASCO Co.) equipped with a Synergi 4 μ fusion-RP column (4.6 × 250 mm; Phenomenex), which was equilibrated with a 5 mM ammonium acetate buffer pH 4.5 to acetonitrile ratio of 97:3 (v/v). HPLC peaks were monitored at 252 nm. The amount of AMP was estimated by calculating the peak area of AMP with a standard calibration curve, which was made by HPLC analysis of the peak area of different concentrations of AMP. Accession codes: Atomic coordinates and structure factors have been deposited in the Protein Data Bank, www.pdb.org (PDB ID codes: 3WV7 , 3WV8 , 3WV9 , 3WVA , 3WVB and 3WVC ). How to cite this article: Fujishiro, T. et al. Protein-pyridinol thioester precursor for biosynthesis of the organometallic acyl-iron ligand in [Fe]-hydrogenase cofactor. Nat. Commun. 6:6895 doi: 10.1038/ncomms7895 (2015).